CO2controls the oriented growth of metal-organic framework with highly accessible active sites The production of 2D metal-organic frameworks (MOFs) with highly exposed active surfaces is of great importance for catalysis. Here we demonstrate the formation of MOF nanosheets by utilizing CO 2 as a capping agent to control the oriented growth of MOF. This strategy has many advantages over the conventional methods. For example, it is template-free and proceeds at mild temperature (35 °C), CO 2 can be easily removed by depressurization, and the properties of the MOF nanosheets can be well adjusted by changing CO 2 pressure. Such a simple, rapid, efficient and adjustable route produces MOF nanosheets with ultrathin thickness ( ∼ 10 nm), small lateral size ( ∼ 100 nm) and abundant unsaturated coordination metal sites on surfaces. Owing to these unique features, the as-synthesized MOF nanosheets exhibit superior activity for catalyzing the oxidation reactions of alcohols. Metal-organic frameworks (MOFs) are a new type of crystalline porous materials that are self-assembled by the coordination of metal cations/clusters with organic linkers [1] , which have broad applications in gas storage and separation [2] , [3] , [4] , catalysis [5] , sensor [6] , drug delivery [7] , etc. Particularly, MOFs have exhibited promising catalytic potentials towards many kinds of reactions owing to their designable metal-oxo clusters bridging organic linkers, modifiable structure, and intrinsic porosities [8] . However, the catalytic activities of MOFs are still largely restricted for the low-mass permeability, poor conductivity, and blockage of active metal centers by organic ligands [9] . Ultrathinning three-dimensional (3D) MOFs into two-dimensional (2D) MOFs is an effective strategy to acquire high-performance catalysts because of the highly exposed active surfaces, superior electron transfer and facilitated mass transport of 2D MOFs [9] , [10] , [11] , [12] , [13] , [14] , [15] . Up to now, the methods for synthesizing 2D MOFs can be classified into two groups: top-down and bottom-up strategies. The top-down exfoliation approach relies on the disintegration of 3D layered MOF solid [11] , [16] , [17] , [18] , [19] , usually suffering from high-energy consumption, fragmentation and morphological damage and low yields (typically < 15%) [9] , [20] . For the bottom-up strategy, 2D MOFs are synthesized directly from starting materials by solvothermal route using additives (e.g., surfactant, capping molecules, template) to control the oriented MOF growth [21] , [22] , [23] , [24] , [25] . The temperature is high (>80 °C) and the post-processing procedure is complex to remove the solid or liquid additives. It is of great importance to develop facile and efficient method for the synthesis of 2D MOFs, promisingly with highly accessible active sites that are desirable for catalysis. Herein we propose a CO 2 -directed route for synthesizing MOF nanosheets. By utilizing CO 2 as a capping agent for controlling the oriented growth of MOF, the MOF nanosheets with ultrathin thickness, small lateral size and highly accessible active sites were obtained. In comparison with the conventional methods for 2D MOFs synthesis, this strategy has many advantages. First, CO 2 can direct the oriented growth of MOF by adsorbing on the specific facets of MOF crystal, involving no additional template. Second, CO 2 accelerates MOF formation at mild temperature (35 °C). Third, the properties of the as-synthesized 2D MOFs can be well adjusted by changing CO 2 pressure. Fourth, CO 2 can be easily removed by depressurization. Moreover, the CO 2 desorption from MOF creates abundant unsaturated sites on surfaces that are desirable for catalysis. The as-synthesized MOF nanosheets have shown highly efficient and reusable catalysts for oxidation reactions of a series of alcohols. Synthesis and structural characterizations of Cu(BDC) nanosheets For the synthesis of Cu(BDC) (BDC = 1,4-benzenedicarboxylate) nanosheets, CO 2 was charged into the methanol solution of Cu(NO 3 ) 2 ·3H 2 O, terephthalic acid and triethylamine (TEA) at 35 °C until a desired pressure was reached (see device in Supplementary Fig. 1 ). After reaction for a certain time, the solid product was obtained by depressurization and washing. 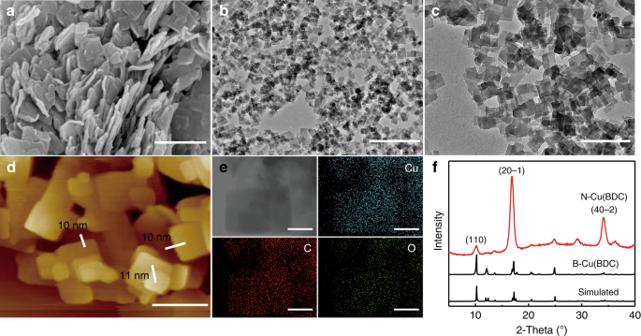Fig. 1: Structural characterizations of N-Cu(BDC). a–eSEM, TEM, AFM images, and EDS mappings of N-Cu(BDC) synthesized in CO2/methanol solution at 7.38 MPa and 35 °C with 0.1 mL of TEA for 24 h;fXRD patterns of N-Cu(BDC), B-Cu(BDC), and simulated XRD pattern of bulk Cu(BDC). Scale bars: 500 nm inaandc, 1 μm inb, 200 nm indand 50 nm ine. Figure 1 shows the characterizations for the product obtained at 7.38 MPa and reaction for 24 h. Scanning electron microscopy (SEM) and transmission electron microscopy (TEM) images show the formation of square nanosheets with edge length of ∼ 120 nm (Fig. 1a–c ). The thickness of nanosheets is ∼ 10 nm, as characterized by atomic force microscope (AFM, Fig. 1d and Supplementary Fig. 2 ). Elemental mapping and energy-dispersive X-ray spectroscopy (EDS) images reveal that Cu, C and O elements distribute evenly in the product (Fig. 1e and Supplementary Fig. 3 ). X-ray diffraction (XRD) pattern mainly exhibits (20-1) and (40-2) crystallographic planes of Cu(BDC) (Fig. 1f ), suggesting that these planes are all perpendicular to the stacking direction of the layers. High-resolution TEM image gives further support that the exposed surface of nanosheet is (20-1) facet (Supplementary Fig. 4 ). In other words, the flat top and bottom surfaces of Cu(BDC) are bounded by (20-1) facets [26] . For comparison, the Cu(BDC) was synthesized by the conventional solvothermal route, which shows cubic crystals with edge dimensions ranging from 0.5 to 10 µm (Supplementary Fig. 5 ). Its XRD pattern and relative intensities of the diffractions match well with the simulated diffractions of bulk Cu(BDC) (Fig. 1f ) [27] . The Cu(BDC) nanosheets synthesized in CO 2 and the bulk Cu(BDC) produced by solvothermal route are denoted as N-Cu(BDC) and B-Cu(BDC), respectively. Fig. 1: Structural characterizations of N-Cu(BDC). a – e SEM, TEM, AFM images, and EDS mappings of N-Cu(BDC) synthesized in CO 2 /methanol solution at 7.38 MPa and 35 °C with 0.1 mL of TEA for 24 h; f XRD patterns of N-Cu(BDC), B-Cu(BDC), and simulated XRD pattern of bulk Cu(BDC). Scale bars: 500 nm in a and c , 1 μm in b , 200 nm in d and 50 nm in e . Full size image Fine structure of N-Cu(BDC) The insightful chemical and structural information of N-Cu(BDC) were investigated by X-ray photoelectron spectroscopy (XPS) (Fig. 2a, b and Supplementary Fig. 6 ). From the high resolution of Cu 2p spectra (Fig. 2a ), the main peak of Cu (934.5 eV) of N-Cu(BDC) shifts to lower binding energy (0.4 eV) as compared with that of B-Cu(BDC). It indicates the presence of low valence state of Cu in N-Cu(BDC) [28] , [29] , [30] , which can be ascribed to the oxygen vacancies or linker missing in framework structure along with the formation of N-Cu(BDC). The O 1s spectrum of N-Cu(BDC) presents two curve-fitted peaks corresponding to two different types of oxygen species (Fig. 2b ). The band at 531.9 eV corresponds to Cu-O species, of which the relative strength is obviously higher than that of B-Cu(BDC). It suggests that more Cu-O clusters are exposed on the surface of Cu(BDC) nanosheet. To further detect the local structure of N-Cu(BDC) at atomic level, the synchrotron X-ray absorption fine structure (XAFS) was determined. For Cu K-edge X-ray absorption near-edge structure (XANES) (Fig. 2c ), the N-Cu(BDC) exhibits similar spectrum features to those of B-Cu(BDC), suggesting that their main structures are the same. The absorption edge of N-Cu(BDC) is at 8989.3 eV, which is between those of B-Cu(BDC) (8989.9 eV) and Cu foil (8979.0 eV). It indicates the existence of Cu δ+ (0 < δ < 2) species in N-Cu(BDC). From extended X-ray absorption fine structure (EXAFS) spectra (Fig. 2d ), the peak centered at 1.53 Å for the N-Cu(BDC) shows an intensity decrease, which further suggests the formed Cu(BDC) nanosheets with lower coordination number [30] . By fitting for EXAFS (Fig. 2e , Supplementary Fig. 7 , and Table 1 ), it is confirmed that the coordination number of Cu is 4.0, which is less than that of B-Cu(BDC) (five oxygen atoms around one Cu atom) [27] . Fourier-transform infrared spectroscopy (FT-IR) proves that carboxylate groups of BDC 2− are coordinated to Cu (II) ions in N-Cu(BDC) (Supplementary Fig. 8 ). Moreover, the absorption of -COO − for N-Cu(BDC) centers at 1628 cm −1 (Fig. 2f ), which is higher than that in B-Cu(BDC) (1624 cm −1 ). It can be ascribed to the more freedom of oxygen atoms in N-Cu(BDC). Fig. 2: Fine structure of N-Cu(BDC). a , b Cu 2p and O 1s XPS spectra of N-Cu(BDC) synthesized in CO 2 /methanol at 7.38 MPa and 35 °C with 0.1 mL of TEA for 24 h and B-Cu(BDC); c XANES spectra at Cu K-edge of B-Cu(BDC), N-Cu(BDC) and Cu foil (inset is the expanded pre-edge region); d EXAFS spectra of B-Cu(BDC) and N-Cu(BDC); e EXAFS fitting curve of N-Cu(BDC); f FT-IR spectra of B-Cu(BDC) and N-Cu(BDC). Full size image Evolution of N-Cu(BDC) with reaction time The formation of N-Cu(BDC) in CO 2 is very interesting and the underlying mechanism was investigated by different experiments. First, the evolution of the N-Cu(BDC) was investigated by varying reaction time, the other conditions being the same with those above. As the reaction time is as short as 20 min, the XRD peak positions and relative intensities of the product agree well with those of the reported Cu(BDC), but the crystallinity is poor (Fig. 3a ). With prolonged reaction time, the crystallinity is enhanced and 24 h is enough to get the well crystallized product. The full-width half-maximum (FWHM) values of (110) peaks of the samples synthesized at different time increase with time, while those of (20-1) peaks decline with reaction time (Fig. 3b ). The relative intensities of (20-1) plane to (110) plane enhance with time (Fig. 3b ). These results indicate that the (20-1) plane grows faster than (110) plane, thus resulting in the formation of Cu(BDC) nanosheets at prolonged reaction time. The sample synthesized at 20 min presents small nanoparticles in average size of 10 nm (Fig. 3c and Supplementary Fig. 9 ). With prolonged reaction time, it changes to the irregular nanosheets with size of ∼ 50 nm at 12 h (Fig. 3c ) and regular nanosheets ( ∼ 120 nm) at 24 and 36 h (Figs. 1c and 3c ). The yields of the materials increase with reaction time and can reach 90% when the reaction time extends to 24 h (Supplementary Fig. 10 ). Fig. 3: Tunability and formation mechanism of N-Cu(BDC). a XRD patterns of the Cu(BDC) synthesized in CO 2 /methanol solution at 7.38 MPa and 35 °C with 0.1 mL of TEA at different time; b Dependence of FWHM of planes and the relative intensity of (20-1) plane to (110) plane ( I 20- 1 /I 110 ) on reaction time; c TEM images of the Cu(BDC) synthesized with time of 20 min, 12 and 36 h; d XRD patterns of the Cu(BDC) synthesized in CO 2 /methanol solution at 35 °C and 24 h with 0.1 mL of TEA at different pressures; e Dependence of the relative intensity of (20-1) plane to (110) plane ( I 20-1 / I 110 ) and the yield of Cu(BDC) on pressure; f TEM images of Cu(BDC) synthesized at 3.40, 6.40 and 8.60 MPa, respectively; g Structural units of Cu(BDC) and CO 2 along [20-1] axis; h Structural units of Cu(BDC) and CO 2 along (20-1) plane. Scale bar: 300 nm in c and f . Full size image Effect of CO 2 pressure on N-Cu(BDC) formation The effect of CO 2 pressure on the N-Cu(BDC) formation was investigated by varying pressure. The reaction time was fixed at 24 h. In the absence of CO 2 (at atmospheric pressure), Cu(BDC) could not be formed in pure methanol, suggesting that CO 2 plays a key role on the Cu(BDC) nanosheets formation (Fig. 3d and Supplementary Fig. 11 ). The main peaks in XRD patterns of the products obtained at pressure of 3.40, 6.40, 8.60 and 10.50 MPa match well with those of the simulated XRD of Cu(BDC) (Fig. 3d ), indicating the formation of Cu(BDC) in presence of CO 2 . Obviously, the relative intensity of (20-1) to (110) is dependent of pressure. It increases slowly at initial stage and increases sharply in pressure range of 6.40–7.38 MPa (Fig. 3e ). It means that more CO 2 is favorable for accelerating the growth of (20-1) plane and simultaneously restrains the (110) plane of Cu(BDC). At the same time, the dependence of the Cu(BDC) yield with pressure shows a similar trend to that of the relative intensity of (20-1) plane to (110) plane (Fig. 3e ). From TEM (Fig. 3f and Supplementary Fig. 12 ) and SEM images (Supplementary Figs. 13 and 14 ), it is clear that high-pressure favors the formation of nanosheets. The average sizes of the nanosheets obtained at 7.38, 8.60, and 10.50 MPa are 120, 102, and 96 nm, with thicknesses of 10, 10, and 7 nm, respectively (Supplementary Figs. 15 – 19 ). Evidently, the size of the N-Cu(BDC) decreases with increasing CO 2 pressure. It is known that CO 2 is well solubilized in organic solvent to cause large volume expansion and lowered viscosity, especially at high pressure (Supplementary Fig. 20 ). Therefore, the CO 2 -expanded solution at higher pressure is favorable for producing N-Cu(BDC) with smaller size [31] , [32] , [33] , [34] . Effect of temperature on Cu(BDC) formation To detect the effect of temperature on N-Cu(BDC) formation, the synthesis was also carried out at 25 °C and 45 °C, respectively, while the pressure was fixed at 7.38 MPa. XRD, SEM, and TEM results reveal the formation of Cu(BDC) nanosheets (Supplementary Figs. 21 – 24 ), which have similar size with those synthesized at 35 °C. It means that the size of Cu(BDC) nanosheets is independent of temperature. The yields of Cu(BDC) nanosheets synthesized at 25, 35, and 45 °C are 69%, 90%, and 95%, respectively. Obviously, higher temperature accelerates the production of Cu(BDC) nanosheets. Effects of other factors on Cu(BDC) formation To get more information on the formation mechanism for Cu(BDC) nanosheets, a series of experiments were carried out. First, Ar or N 2 was used as an alternative of CO 2 to synthesize Cu(BDC) in methanol. The gas pressure and reaction time were fixed at 7.30 MPa and 24 h, respectively, the other experimental conditions being the same with above. The results show that Cu(BDC) nanosheets could not be formed by using Ar or N 2 (Supplementary Figs. 25 and 26 ). Second, the Cu(BDC) synthesis was carried out in CO 2 /acetonitrile and CO 2 /ethanol solutions at 7.38 MPa and 35 °C, respectively. The Cu(BDC) nanosheets that are similar to those formed in CO 2 /methanol solution were obtained (Supplementary Figs. 27 and 28 ). It proves that it is indeed CO 2 that dominates the formation of Cu(BDC) nanosheets. Third, to detect whether the carbonation of CO 2 in water has an effect on N-Cu(BDC) formation, the MOF synthesis was carried out in Na 2 CO 3 /methanol and NaHCO 3 /methanol solutions (without CO 2 ), respectively. The obtained products present large irregular agglomerates (Supplementary Figs. 29 and 30 ). Therefore, the effect of CO 2 ionization in water on the N-Cu(BDC) formation can be ruled out. Fourth, the effect of TEA dosage on the formation of N-Cu(BDC) in CO 2 /methanol solution was studied. The pressure and temperature were fixed at 7.38 MPa and 35 °C, respectively. It was found that the enough amount of TEA, which plays a role for H 2 BDC deprotonation, is needed for accelerating the reaction between Cu 2+ and the deprotonated BDC 2− to form framework building blocks and the further nanosheet formation (Supplementary Figs. 31 and 32 ). Density functional theory (DFT) calculations To further understand the underlying mechanism for the CO 2 -produced Cu(BDC) nanosheets, DFT calculations were performed. The interaction distance between O in CO 2 and Cu ion along [20-1] axis was calculated to be 2.641 Å, while that along (20-1) plane is 2.950 Å belonging to non-bonded interaction (Fig. 3g , h). It indicates that CO 2 is more easily adsorbed on the (20-1) crystal facet, so as to forbid the stacking of (20-1) crystal facets along [20-1] axis. (20-1) plane is the dominantly exposed crystal facets and CO 2 has no effect on the coordination between organic ligands and Cu 2+ along (20-1) plane (Supplementary Fig. 33 ). It is worth noting that the interactions of Cu(BDC) with methanol along (20-1) plane and [20-1] axis are almost equivalent (Supplementary Fig. 34 ). Therefore, it can be understood that pure methanol has no effect to direct the 2D growth of Cu(BDC) and cannot produce nanosheets (Supplementary Fig. 11 ). Formation mechanism of N-Cu(BDC) Based on the above results, a possible mechanism for the formation of Cu(BDC) nanosheets by CO 2 is proposed (Supplementary Fig. 35 ). First, Cu 2+ react with the deprotonated BDC 2− by TEA to structure the nanosized framework building blocks. Subsequently, CO 2 molecule interacts with Cu 2+ on (20-1) plane, which forbids the stacking of (20-1) crystal facets along [20-1] axis. The viscosity-lowering effect caused by CO 2 would promote mass transfer and accelerate the formation of MOF nanocrystals. After reaction, CO 2 is released by depressurization, during which the desorption of CO 2 leaves abundant uncoordinated sites on the surface of Cu(BDC) nanosheets. The as-synthesized N-Cu(BDC) has a much improved CO 2 adsorption ability than the bulk Cu(BDC) produced in pure methanol (Supplementary Fig. 36 ). The above result that high CO 2 pressure benefits to the formation of Cu(BDC) nanosheets can be well understood (Fig. 3d–f ). At low pressure, the amount of CO 2 solubilized in reaction system is small, as well as the CO 2 adsorbed on (20-1) crystal facets. Consequently, CO 2 cannot control the oriented growth of Cu(BDC) effectively. The massive dissolution of CO 2 in reaction system makes the sufficient adsorption of CO 2 on (20-1) crystal facets when the pressure reaches 7.38 MPa, so as to direct the 2D growth of Cu(BDC) crystal. At the same time, the viscosity-lowering effect caused by CO 2 is more obvious at higher pressure, which favors the production of Cu(BDC) nanosheets with larger yield. Catalytic activities of N-Cu(BDC) The N-Cu(BDC) was used to catalyze the oxidation of benzyl alcohol to benzaldehyde (Fig. 4a ), which is an important reaction both in organic synthesis and chemical industry [35] , [36] , [37] . The catalytic reaction was performed under 75 °C, using 2,2,6,6-teramethyl-piperidine-1-oxyl (TEMPO) as a co-catalyst, Na 2 CO 3 as base, oxygen as oxidant and N,N-dimethylformamide (DMF) as solvent. First of all, a control experiment for benzyl alcohol oxidation in the presence of only TEMPO (without N-Cu(BDC)) was carried out, which shows that benzyl alcohol cannot be converted in 2.5 h. With the addition of N-Cu(BDC), the conversion of benzyl alcohol to benzaldehyde reaches 99% at 2.5 h, with selectivity of >99% (Fig. 4b ). In sharp contrast, the yield of benzaldehyde is only 49% after a reaction time of 2.5 h as catalyzed by B-Cu(BDC) at the same conditions. 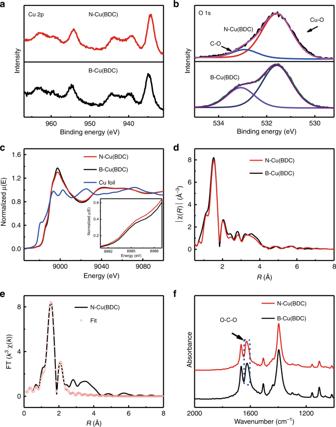Fig. 2: Fine structure of N-Cu(BDC). a,bCu 2p and O 1s XPS spectra of N-Cu(BDC) synthesized in CO2/methanol at 7.38 MPa and 35 °C with 0.1 mL of TEA for 24 h and B-Cu(BDC);cXANES spectra at Cu K-edge of B-Cu(BDC), N-Cu(BDC) and Cu foil (inset is the expanded pre-edge region);dEXAFS spectra of B-Cu(BDC) and N-Cu(BDC);eEXAFS fitting curve of N-Cu(BDC);fFT-IR spectra of B-Cu(BDC) and N-Cu(BDC). The catalytic activity of N-Cu(BDC) for the oxidation of benzyl alcohol to benzaldehyde is also higher than the mesoporous Cu 3 (BTC) 2 under similar reaction conditions [34] (Supplementary Table 2 ). After reaction, the N-Cu(BDC) was recovered and its reusability for the reaction was tested using benzyl alcohol as a model substrate. The conversion of benzyl alcohol remains unchanged at the 5th run for catalysis (Supplementary Fig. 37 ). No obvious difference was observed for the XRD pattern and TEM images of fresh Cu(BDC) and that after reused for five runs (Supplementary Fig. 38 ), indicating the well preserved structural integrity of N-Cu(BDC) catalyst. Inductively coupled plasma atomic emission spectrometer (ICP-AES) was used to determine whether there was Cu leached to DMF after reaction for five runs. No copper ions were detected, confirming the stability of N-Cu(BDC) for the oxidation reaction in DMF. Fig. 4: Catalytic activities of N-Cu(BDC) and B-Cu(BDC). a Aerobic oxidation of benzyl alcohol on N-Cu(BDC) synthesized in CO 2 /methanol solution at 7.38 MPa and 35 °C with 0.1 mL of TEA for 24 h; b – e Time conversion plot for the aerobic oxidation of benzyl alcohol, 3-nitrobenzyl alcohol, 4-methylbenzyl alcohol, and cinnamyl alcohol to corresponding products catalyzed by N-Cu(BDC) and B-Cu(BDC), respectively. Full size image The catalytic activities of the as-synthesized N-Cu(BDC) were tested for the aerobic oxidation of various alcohols (Fig. 4c–e ). 3-nitrobenzyl alcohol, 4-methylbenzyl alcohol and cinnamyl alcohol converted completely to the corresponding aldehydes in 3, 2, and 2 h, respectively. In contrast, the aldehyde yields catalyzed by B-Cu(BDC) only reach 51%, 38%, and 75% for these three alcohols at reaction time of 3, 2, and 2 h, respectively. The aerobic oxidations of furfuryl alcohol, 2-naphthalenemethanol, 1-phenylethanol, and 1-(4-methoxyphenyl)ethanol as catalyzed by N-Cu(BDC) were also studied. 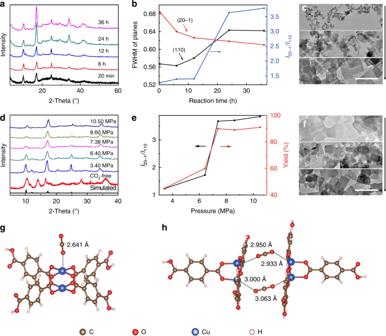Fig. 3: Tunability and formation mechanism of N-Cu(BDC). aXRD patterns of the Cu(BDC) synthesized in CO2/methanol solution at 7.38 MPa and 35 °C with 0.1 mL of TEA at different time;bDependence of FWHM of planes and the relative intensity of (20-1) plane to (110) plane (I20-1/I110) on reaction time;cTEM images of the Cu(BDC) synthesized with time of 20 min, 12 and 36 h;dXRD patterns of the Cu(BDC) synthesized in CO2/methanol solution at 35 °C and 24 h with 0.1 mL of TEA at different pressures;eDependence of the relative intensity of (20-1) plane to (110) plane (I20-1/I110) and the yield of Cu(BDC) on pressure;fTEM images of Cu(BDC) synthesized at 3.40, 6.40 and 8.60 MPa, respectively;gStructural units of Cu(BDC) and CO2along [20-1] axis;hStructural units of Cu(BDC) and CO2along (20-1) plane. Scale bar: 300 nm incandf. 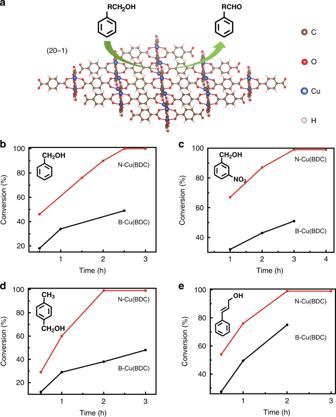Fig. 4: Catalytic activities of N-Cu(BDC) and B-Cu(BDC). aAerobic oxidation of benzyl alcohol on N-Cu(BDC) synthesized in CO2/methanol solution at 7.38 MPa and 35 °C with 0.1 mL of TEA for 24 h;b–eTime conversion plot for the aerobic oxidation of benzyl alcohol, 3-nitrobenzyl alcohol, 4-methylbenzyl alcohol, and cinnamyl alcohol to corresponding products catalyzed by N-Cu(BDC) and B-Cu(BDC), respectively. At 2.5 h, these alcohols can be converted to their corresponding aldehydes with yields of 70%, 89%, 44%, and 40%, respectively (Supplementary Table 3 ), which are all higher than those catalyzed by the reported Cu 3 (BTC) 2 at similar conditions [38] . Moreover, the catalytic activities of Cu(BDC) catalysts synthesized in CO 2 /methanol solutions at different CO 2 pressures and 35 °C for catalyzing the oxidation of benzyl alcohol to benzaldehyde were studied. The reaction conditions were the same with those above. As catalyzed by Cu(BDC) synthesized at 3.40 and 6.40 MPa, the yields of benzaldehyde are 62% and 85%, respectively, while the yields of benzaldehyde catalyzed by Cu(BDC) synthesized at pressures higher than 7.38 MPa is 99% (Supplementary Table 2 ). It is obvious that the Cu(BDC) synthesized at higher pressure is more active, which can be attributed to its smaller size and more exposed active sites for catalysis [39] . The high catalytic activity of the N-Cu(BDC) synthesized in this work can be attributed to their smaller particle size and more unsaturated metal sites than that synthesized by hydrothermal route. First, the N-Cu(BDC) synthesized by CO 2 has nanometer sizes in all the three dimensions, which is favorable to increasing the density of catalytic active sites. Second, the N-Cu(BDC) synthesized by CO 2 has abundant unsaturated coordination Cu sites on surfaces that are available for catalysis [40] , [41] , [42] , which are superior to the dormant and fully coordinated framework metal ions of MOFs that are unavailable for catalysis. Owing to these unique features, the as-synthesized N-Cu(BDC) exhibits greatly enhanced activity for catalyzing the oxidation reactions of alcohols as compared with B-Cu(BDC). The versatility of the CO 2 -directed route for the formation of other MOF nanosheets was investigated. The nanosheets of MOFs with different metal ions and organic ligands, i.e., Co(BDC), Cu(1,4-NDC) (1,4-NDC = 1,4-naphtalenedicarboxylate), bi-metal (Co, Ni)(BDC) were successfully synthesized (Supplementary Figs. 39 – 51 ). Moreover, the CO 2 -directed route can be applied to the large-scale synthesis of Cu(BDC) nanosheets (Supplementary Figs. 52 and 53 ). In summary, we propose a CO 2 -directed route for controlling the oriented growth of MOF. This strategy produces MOF nanosheets with ultrathin thickness ( ∼ 10 nm), ultra-small lateral size ( ∼ 100 nm) and abundant unsaturated coordination metal sites on the surface of nanosheets. These combined features confer the as-synthesized MOF nanosheets many advantages for catalyzing chemical reactions, particularly facilitating the approach of reactant molecules to catalytically active sites. The proposed CO 2 method is facile, rapid, adjustable, high-yielding, low-energy and environmentally benign for MOF material synthesis. We anticipate that it could be applied to the fabrication of other MOFs and MOF-based materials with desirable structures and functions. Materials Terephthalic acid (H 2 BDC, 99% purity), methyl sulfoxide-d6 (99.8% atom% D purity), cinnamyl alcohol (98% purity), 3-nitrobenzyl alcohol (>99% purity), 4-methylbenzyl alcohol (98% purity), and TEMPO (98% purity) were supplied by Beijing InnoChem Science & Technology Co., Ltd. CO 2 ( >99.95% purity), water, N 2 ( >99.95% purity), Ar (>99.999% purity), and O 2 (99.99% purity) were purchased from Beijing Analysis Instrument Factory. TEA (A. R. grade), ethanol (A. R. grade), methanol (A. R. grade), DMF (A. R. grade), acetonitrile (A. R. grade), Na 2 CO 3 (A. R. grade), and NaHCO 3 (A. R. grade) were supplied by Beijing Chemical Works. CoCl 2 ·6H 2 O (A. R. grade), Cu(NO 3 ) 2 ·3H 2 O (A. R. grade), and NiCl 2 ·6H 2 O (A. R. grade) were brought from China National Medicines Co., Ltd. 1,4-Naphthalenedicarboxylic acid (H 2 NDC, 99% purity), 2-naphthalenemethanol (98% purity), 1-phenylethanol (97% purity), 1-(4-methoxyphenyl)ethanol (95% purity), and furfuryl alcohol (98% purity) were purchased from J&K Scientific Co., Ltd. Benzyl alcohol was supplied by Alfa Aesar China Co., Ltd. All these materials were used directly without further purification. Cu(BDC) synthesis For a typical experiment, Cu(NO 3 ) 2 ·3H 2 O (0.0180 g), H 2 BDC (0.0170 g), TEA (0.1 mL) and methanol (5 mL) were added into autoclave. Then CO 2 was charged into the autoclave under stirring to the desired pressure for 24 h at 35 °C. The precipitate was collected, washed by DMF and ethanol twice and dried at 80 °C in vacuum for 8 h. A series of control experiments were carried out. First, N 2 or Ar was used as an alternative of CO 2 for Cu(BDC) synthesis, while the other conditions were the same with those above. Second, Cu(BDC) was synthesized in CO 2 /ethanol and CO 2 /acetonitrile solutions, respectively, the other conditions being the same with those above for the synthesis in CO 2 /methanol solution (35 °C and 7.38 MPa). Third, the Cu(BDC) synthesis was conducted in NaHCO 3 /methanol and Na 2 CO 3 /methanol solution (without CO 2 ), respectively. The amount of NaHCO 3 or Na 2 CO 3 was 20 mg, while the dosages of other reagents were the same with those above for the synthesis in CO 2 /methanol solution. Bulk Cu(BDC) synthesis Bulk Cu(BDC) was synthesized following the hydrothermal synthesis described by Carson [27] . 0.5000 g of Cu(NO 3 ) 2 ·3H 2 O, 0.3500 g of H 2 BDC and 43 mL of DMF were mixed in a 100 mL round-bottom flask and refluxed at 100 °C for 24 h. The resulting powder was collected by centrifugation at 10,000 rpm and the solid was consecutively washed with DMF (20 mL each step) and ethanol (20 mL each step) for three times, respectively. The product was obtained after drying at 80 °C in vacuum for 8 h. Co(BDC) nanosheets synthesis CoCl 2 ·6H 2 O (0.0108 g) and H 2 BDC (0.0100 g) were dissolved into 4 mL DMF mixed with 0.25 mL water and 0.25 mL ethanol. The above solution was stirred for 30 min, followed by the addition of 0.1 mL TEA. Then CO 2 was charged into the autoclave under stirring. The mixture was stirred at 7.38 MPa and 35 °C for 24 h. The precipitate was washed by DMF and ethanol twice and dried at 80 °C in vacuum for 8 h. Cu(1,4-NDC) nanosheets synthesis Cu(NO 3 ) 2 ·3H 2 O (0.0180 g), H 2 NDC (0.0210 g), methanol (5 mL) and TEA (0.1 mL) were added into autoclave. CO 2 was charged into the autoclave under stirring. Then the mixture was stirred at 7.38 MPa and 35 °C for 24 h. The precipitate was collected, washed by DMF and ethanol twice and dried at 80 °C in vacuum for 8 h. (Co, Ni)(BDC) nanosheets synthesis CoCl 2 ·6H 2 O (0.0108 g), NiCl 2 ·6H 2 O (0.0108 g) and H 2 BDC (0.0180 g) were dissolved into 4 mL DMF mixed with 0.25 mL water and 0.25 mL ethanol. The above solution was stirred for 30 min, followed by the addition of 0.1 mL TEA. Then CO 2 was charged into the autoclave under stirring. The mixture was stirred at 7.38 MPa and 35 °C for 24 h. The precipitate was washed by DMF and ethanol twice and dried at 80 °C in vacuum for 8 h. Characterizations The morphologies of the as-synthesized materials were characterized by SEM (HITACHI S-4800) and TEM (JEOL-1010) operated at 100 kV. High-resolution TEM was characterized by Cryo-EM (Thermoscientific themis 300). XRD was performed on a Rigaku D/max-2500 diffractometer with Cu Kα radiation ( λ = 1.5418 Å) at 40 kV and 200 mA. XPS was determined by VG Scientific ESCALab220i-XL spectrometer using Al Ka radiation. FT-IR spectra of the samples were performed on a Bruker Tensor 27 spectrometer. Liquid 1 H NMR spectra were recorded on Bruker 400 spectrometer. The X-ray absorption spectroscopy experiment was carried out at Beamline 1W2B at Beijing Synchrotron Radiation Facility. Computational method The DFT calculations were performed through DMol3 package [43] , [44] , [45] . The exchange-correlation energy was calculated within the generalized gradient approximation using the function proposed by Perdew and Wang (PW91) with dispersion correction (DFT-D). Structural optimizations were obtained on the basis of the convergence criterion in which SCF tolerance was 1.0 × 10 −6 Ha, while the convergence tolerances of energy, maximum force, and maximum displacement were 1.0 × 10 −5 Ha, 2.0 × 10 −3 Ha Å −1 , and 5.0 × 10 −3 Å, correspondingly. A Fermi smearing of 2.0 × 10 −3 Ha and a cutoff radius of 5.5 Å were used to accelerate convergence. The double numerical plus polarization (DNP) basis sets with effective core potential were employed to express atomic potentials. The adsorption energy between the segment of structural units of Cu-MOF and adsorbed gas (CO 2 ) is determined using ∆ E = E (A n B m ) – n * E (A) – m * E (B), where E (A n B m ), E (A), and E (B) denote the total energies of the segment of A n B m , A, and B, respectively [46] , [47] . Catalysis study The procedure was similar to that reported by Dhakshinamoorthy and co-workers [38] . Benzyl alcohol 20 mg, catalyst 30 mg, TEMPO 14 mg, Na 2 CO 3 20 mg, and 1 mL DMF were added in a 5 mL flask. The reaction temperature was kept at 75 °C and stirred at oxygen atmosphere. After the desired time, the heterogeneous mixture was cooled and centrifuged. The liquid mixture was analyzed by 1 H-NMR method, which was conducted on a Bruker Avance III 400 HD spectrometer in DMSO-d6. For the reusability study, the N-Cu(BDC) catalyst after 2.5 h of reaction was recovered by centrifugation, washed with ethanol and dried under vacuum. Then the catalyst was added into 1 mL DMF containing TEMPO (14 mg), Na 2 CO 3 (20 mg) and benzyl alcohol (20 mg) for a consecutive run. ICP-AES (VISTA-MPX) was used to determine whether there was Cu leached to DMF after reaction for five runs.